Dynamical preparation of Floquet Chern insulators Realizing topological insulators is of great current interest because of their remarkable properties and possible future applications. There are recent proposals based on Floquet analyses that one can generate topologically non-trivial insulators by periodically driving topologically trivial ones. Here we address what happens if one follows the dynamics in such systems. Specifically, we present an exact study of the time evolution of a graphene-like system subjected to a circularly polarized electric field. We prove that for infinite (translationally invariant) systems the Chern number is conserved under unitary evolution. For systems with boundaries, on the other hand, we show that a properly defined topological invariant, the Bott index, can change. Hence, it should be possible to experimentally prepare topological states starting from non-topological ones. We show that the chirality of the edge current in such systems can be controlled by adjusting the filling. Topological and Chern insulators are fascinating phases of quantum matter that are qualitatively different from conventional insulators and semiconductors [1] , [2] . They are characterized by a gap in the bulk and have topologically protected gapless excitations at the boundary [3] , [4] . Topological phases fall outside the Landau–Ginsburg (effective) theory of spontaneous symmetry breaking and are characterized by bulk topological invariants, such as the Chern number [5] , which can be interpreted as non-local order parameters. Recently, it has been proposed that time-periodic perturbations can induce topological properties in otherwise non-topological materials, opening the exciting possibility of studying non-equilibrium topological transitions [6] , [7] , [8] . The link between topology and time-periodic driving can be established via the Floquet theorem [9] , [10] , [11] , [12] , which is very similar to Bloch’s theorem [13] . The Floquet theorem states that the evolution operator of any system described by a time periodic Hamiltonian H ( t )= H ( T + t ) can be factorized as where P ( t , 0)= P ( t + T , 0) is a unitary periodic operator and H F [0] is the time-independent Floquet Hamiltonian. Being time independent, the Floquet Hamiltonian can be characterized using standard concepts developed for undriven situations. For example, the Floquet Hamiltonian is considered topological if the Chern number of the Floquet bands is non-zero [8] . As noted in ref. 14 , this characterization is incomplete since it ignores the properties encoded into the operator P . Moreover, periodically driven systems are manifestly out of equilibrium and the topological properties of the time-evolving state do not need to reflect the topology of the underlying Floquet Hamiltonian. Here we extend the topological characterization above to isolated, thermodynamically large, out-of-equilibrium systems. In particular, we address what should happen in an experiment on an isolated system when one turns on the periodic driving using linear ramps. For infinite (translationally invariant) systems, in the absence of dissipation, we prove a no-go theorem. We show that the Chern number is conserved under unitary evolution. On the other hand, for systems with boundaries, we show that a properly defined topological invariant, the Bott index [15] , can change. Hence, it is possible to dynamically prepare a topological wavefunction starting from a non-topological one via unitary evolution. Model We consider the following Hamiltonian (or a unitary equivalent): where H S is time independent, H 1 ( t ) is time periodic with period T and the amplitude f ( t ) is given by We restrict our analysis to non-interacting fermionic Hamiltonians, for which a complete characterization of the (equilibrium) topological phases exists [16] . We take the initial state to be the ground state of the static Hamiltonian H S . At time t >0, the time-dependent wavefunction is . We are interested in situations in which the undriven system is described by a topologically trivial Hamiltonian H S and the driving is such that the Floquet Hamiltonian H F is topologically non-trivial. We focus on spinless fermions in a honeycomb lattice with nearest-neighbour hopping J and a staggered sublattice potential Δ subjected to a circularly polarized electric field [6] , [7] . In the electromagnetic gauge, in which the vector potential is zero, the time-dependent Hamiltonian is given by equation (2) with where the sum in H S extends over nearest-neighbour sites, α ∈ {1, 2} indicates the sublattice and , respectively, are the site number operators, is the electrostatic potential energy, and e is the electric charge. We work in the high-frequency limit in which the driving frequency is larger than the single-particle bandwidth [17] , that is, . In this limit, there is no ambiguity in the ordering of the Floquet quasi-energies and therefore the ground state of the Floquet Hamiltonian is well defined. Moreover, to obtain a non-trivial high-frequency limit, we scale the electric field with the frequency of the driving [18] , where a is the lattice spacing. Our parameters are: and are chosen so that the (effective) Floquet Hamiltonian H F is topological (results for other value of K are presented only in Fig. 4 ). The staggered sublattice potential Δ is introduced to make direct connection with the experiment in ref. 17 , and to ensure that the edge modes that are not topological in nature are gapped out. The period of the driving is T =2 π /Ω and we consider ramping times . We stress that this choice of parameters is relevant for the recent experimental realization of the Haldane model in cold atoms [17] . In ref. 17 , =20 ms and 1/ T =Ω/(2 π )=4 kHz so that =80. However, the loading procedure there was more complex than the linear ramp considered here. Figure 4: Scaling analysis of the critical fields at which the systems become topological. ( a ) The critical electric field E c at which the Floquet Hamiltonian becomes topological decreases exponentially with the linear size of the system, , and approaches E c =3.47 in the thermodynamic limit. This value is compatible with the value at which the translationally invariant system becomes topological (see b ). 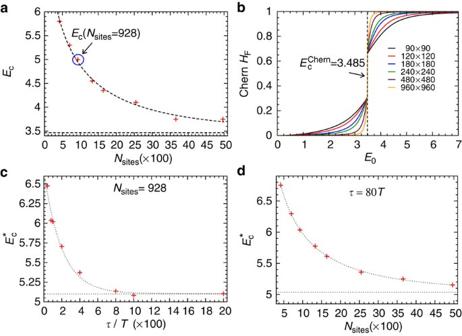Figure 4: Scaling analysis of the critical fields at which the systems become topological. (a) The critical electric fieldEcat which the Floquet Hamiltonian becomes topological decreases exponentially with the linear size of the system,, and approachesEc=3.47 in the thermodynamic limit. This value is compatible with the value at which the translationally invariant system becomes topological (seeb). (b) The equilibrium Chern number of the translationally invariant system jumps discontinuously at=3.485 indicating that, forE>, the translationally invariant system becomes topological. (c) For a fixed system size (Nsites=928), the value of the electric fieldat which the wavefunction becomes topological decreases exponentially with/Tand approaches=5.10 as/T→∞. This value is compatible with the value at whichHFbecomes topological forNsites=928 (see the point indicated by an arrow ina). (d) For fixed ramp time (=80T), critical fieldat which the wavefunction becomes topological decreases exponentially withLand approaches=5.04 in the thermodynamic limit. ( b ) The equilibrium Chern number of the translationally invariant system jumps discontinuously at =3.485 indicating that, for E > , the translationally invariant system becomes topological. ( c ) For a fixed system size ( N sites =928), the value of the electric field at which the wavefunction becomes topological decreases exponentially with / T and approaches =5.10 as / T →∞. This value is compatible with the value at which H F becomes topological for N sites =928 (see the point indicated by an arrow in a ). ( d ) For fixed ramp time ( =80 T ), critical field at which the wavefunction becomes topological decreases exponentially with L and approaches =5.04 in the thermodynamic limit. Full size image Translationally invariant system We first consider the translationally invariant (infinite) system. In this case, it is convenient to work in the electromagnetic gauge in which the electric field is represented via the vector potential, that is, E ( t )=− t A ( t ), as this gauge choice does not break translational invariance. By going to momentum space the system can be mapped, at half filling, onto a collection of independent pseudo spin- . The Hamiltonian and the density matrix are (we take in what follows): Here, 1 2 × 2 is the 2 × 2 identity matrix, σ are the Pauli matrices and S k and B k are three-dimensional time-dependent vector fields defined in the two-dimensional Brillouin zone (see Supplementary Fig. 1a ). For a pure state, the vector S k has unit length and the Chern number (Ch) of the state is simply the number of wrappings of the pseudo-spin configuration around the Bloch sphere [5] : Here the integral extends over the Brillouin zone. In the ground state, the pseudo-spin configuration is parallel to the pseudo magnetic field, that is, . This does not need to be the case out of equilibrium, where S k and B k are in general not parallel to each other. The exact equation of motion is: which is simply the precession of the pseudo spin S k around the pseudo magnetic field B k . With this mapping, the ground states and obtained by filling the valence bands of H S and H F are represented by the pseudo-spin configurations and , respectively. We note that this mapping is valid for any two-band model at half filling. The explicit form of B k ( t ) in the case of graphene subject to the circularly polarized electric field is given in the Supplementary Note 1 . For the parameters chosen (equation (5)) these ground states have different topology: does not wrap around the Bloch sphere (Ch=0) while does (Ch=−1) (see Fig. 1a,b ). 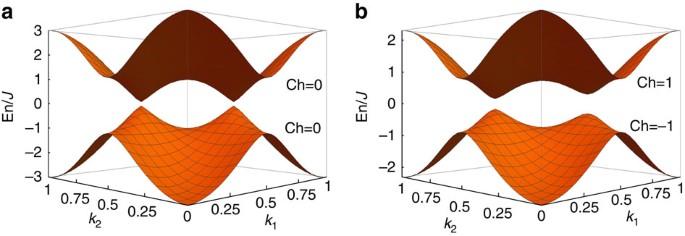This implies that there is at least one k -point in the Brillouin zone for which the vectors and point in opposite directions ( Supplementary Fig. Figure 1: Energy ‘En’ band structure of the infinite, translationally invariant system in units of the hoppingJ. (a) The band structure ofHShas a gap of size Δ at the two Dirac points and the Chern number of each band is zero. (b) The band structure ofHFhas a gap of size∼0.30Jand∼0.16Jat the two Dirac points (the two gaps become equal only when Δ=0), and the Chern number of the bands is +1 (top) and −1 (bottom). Moreover the bandwidth is renormalized from 6Jto 6J(whereis the zeroth Bessel function of first kind andKis defined in equation (5)). 1b and Supplementary Note 2 ) and, as a result, the overlap of the ground states is identically zero: Figure 1: Energy ‘En’ band structure of the infinite, translationally invariant system in units of the hopping J . ( a ) The band structure of H S has a gap of size Δ at the two Dirac points and the Chern number of each band is zero. ( b ) The band structure of H F has a gap of size ∼ 0.30 J and ∼ 0.16 J at the two Dirac points (the two gaps become equal only when Δ=0), and the Chern number of the bands is +1 (top) and −1 (bottom). Moreover the bandwidth is renormalized from 6 J to 6 J (where is the zeroth Bessel function of first kind and K is defined in equation (5)). Full size image We can now consider the dynamical process by which the periodic driving is turned on. In principle, the Chern number inherits a time dependence from the time dependence of the pseudo-spin configuration S ( t ) obtained by integrating the equation of motion (8) subject to the initial condition . However, a straightforward calculation shows that this is not the case. This follows from the fact that t Ch can be written as: If S k ( t ) and B k ( t ) are sufficiently smooth vector fields in the Brillouin zone then it follows that the expression above is identically zero (see Methods). From equation (8) one can see that an initially smooth pseudo-spin configuration S k ( t ) remains smooth under a smooth pseudo magnetic field B k ( t ). We can therefore formulate a no-go theorem as follows: ‘If the initial pseudo-spin configuration is smooth (at least ) in the Brillouin zone and the pseudo magnetic field is smooth (at least ), then the Chern number is conserved under the unitary evolution generated by the pseudo magnetic field.’ We note that this theorem is valid for any two-band model at half filling for which the mapping in equation (6) applies. Moreover the theorem holds even for time-dependent Hamiltonians and/or gapless Hamiltonians, as long as B k ( t ) is in the Brillouin zone for all times. Finally smoothness in time is not required, that is, our results also apply to sudden quenches for which the conservation of the Chern number has been noted before in various contexts [19] , [20] , [21] . We should stress that the smoothness of B k ( t ) in k is guaranteed by the locality of the H ( t ) in real space, that is, B k ( t ) can become singular in k only if the Hamiltonian H ( t ) includes infinite range hopping in real space, and it is therefore not very restrictive. For example, the band structure of graphene is singular at the two Dirac points, but the pseudo magnetic field configuration: is analytic in the Brillouin zone and satisfies the condition of the theorem. The no-go theorem opens the question of whether it is experimentally possible to prepare a topologically non-trivial state by driving a topologically trivial one. System with boundaries Experimental systems have boundaries, so here we address what happens when translational invariance is broken. We consider a finite, isolated system (such that the dynamics is unitary) with open boundary conditions (see Fig. 2a ). To characterize the topological properties of systems with broken translational symmetry one cannot rely on the Chern number. 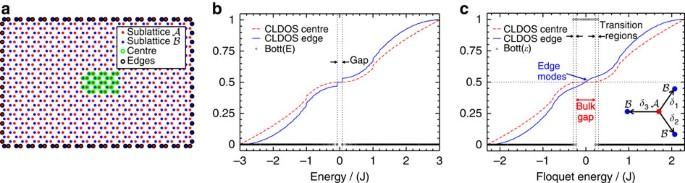We use two complementary indicators: the cumulative local density of states ; and the Bott index [15] . Figure 2: Geometry and indicators for the system with boundaries. (a) One of the patch geometries considered. It contains a total of 928 lattice sites evenly divided into the(red dots) and(blue dots) sublattices. The green and black circles indicate the sites defined as the centre and the edges, respectively. These sites are used to compute the CLDOS. (b) The CLDOS ofHSis flat aroundɛ=0 indicating a gap. The Bott index is identically zero for all energies. (c) ForHF, the CLDOS at the edges (at the centre) has a finite (zero) slope aboutɛ=0. This indicates the presence of edge states inside the bulk gap. Moreover, the Bott index for energies within the bulk gap is +1 indicating that the system is topological. Inset incshows a site in sublatticeand its three nearest neighbours. The nearest-neighbour vectors are:,δ3=a(−1, 0). Figure 2: Geometry and indicators for the system with boundaries. ( a ) One of the patch geometries considered. It contains a total of 928 lattice sites evenly divided into the (red dots) and (blue dots) sublattices. The green and black circles indicate the sites defined as the centre and the edges, respectively. These sites are used to compute the CLDOS. ( b ) The CLDOS of H S is flat around ɛ =0 indicating a gap. The Bott index is identically zero for all energies. ( c ) For H F , the CLDOS at the edges (at the centre) has a finite (zero) slope about ɛ =0. This indicates the presence of edge states inside the bulk gap. Moreover, the Bott index for energies within the bulk gap is +1 indicating that the system is topological. Inset in c shows a site in sublattice and its three nearest neighbours. The nearest-neighbour vectors are: , δ 3 = a (−1, 0). Full size image The Bott index is a topological invariant that can be thought as the generalization of the Chern number for finite, non-translationally invariant systems. Some remarkable properties of the Bott index are: it is computed directly in real space; it is quantized for finite systems; and it can be defined in a patch geometry. This is in contrast to the Chern number that is computed by integrating the partial derivatives of the wavefunction over a two-dimensional torus, is generically non-quantized when the integration is replaced by a discrete sum and cannot be defined in a patch geometry. In ref. 15 , the Bott index was introduced for finite, disordered two-dimensional systems with periodic boundary conditions (that is, on a torus), but it can be straightforwardly generalized to other geometries (see Methods). In equilibrium, the Bott index is a function of the energy ɛ . It is computed by projecting special matrices (see Methods) onto the subspaces spanned by the eigenstates of the Hamiltonian with energies ɛ ′< ɛ . This definition assumes that the eigenstates with energy ɛ ′< ɛ are fully occupied while the eigenstates with energies ɛ ′> ɛ are empty. We have extended the Bott index definition to arbitrary sample geometries and non-equilibrium situations by taking into account the non-equilibrium character of the wavefunction (see Methods). The numerical evidence gathered in this work strongly suggests that this generalized Bott index is a function of time and is quantized. However, these properties have not been proven rigorously. In Fig. 2a , we show one of the patch geometries considered and indicate the edge and bulk sites that have been used to compute the CLDOS. In Fig. 2b,c , we show the CLDOS and the equilibrium Bott index for the static Hamiltonian H S and the Floquet Hamiltonian H F , respectively. We stress that the Floquet Hamiltonian is computed exactly (see Methods). The CLDOS( ɛ ) of H S (both at the centre of the sample and along the edges) has a plateau around ɛ =0 signifying that there are no states at ɛ =0, that is, the system is gapped. Moreover, the Bott index is identically zero indicating that both H S and its ground state are topologically trivial. On the contrary, H F has edge states inside the bulk gap, as shown by the finite (zero) slope of the CLDOS at the edge (centre) for ɛ ≈0. The existence of topologically protected edge modes is confirmed by the Bott index. In fact, in equilibrium, the Bott index at energy ɛ, i.e. Bott( ɛ ), is equal to the number of edge states at that energy. As one can see in Fig. 2c , , indicating that the ground state of H F at half filling ( ɛ =0) is topologically non-trivial. To study the adiabatic turning on of the periodic driving, we solve the time-dependent Schrödinger equation [22] , [23] subject to the initial condition (see Methods). At stroboscopic times t n = nT during the time evolution, we monitor the Bott index and the overlaps of with both the initial state and the Floquet ground state: Their behaviour, for a system of size N sites =928 and ramping time =80 T , is shown in Fig. 3 . 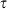One can see that overlap with the initial state decays to zero rapidly while the overlap with the ground state of the Floquet Hamiltonian increases. Figure 3: Dynamical ramp with=80TandNsites=928 in a system with boundaries. (Main) The evolution, at stroboscopic timestn=nT, of the Bott index and the overlapsand. Forξ=t−>0, the electric field is fully on. The overlapis a non-monotonic function oftn=nT. (Inset) The overlap at the end of the dynamical ramp tends to increase with increasing. For t n = nT > , the electric field has reached its final value and the overlap with becomes independent on n since is an eigenstate of the evolution operator over a period: Figure 3: Dynamical ramp with =80 T and N sites =928 in a system with boundaries. (Main) The evolution, at stroboscopic times t n = nT , of the Bott index and the overlaps and . For ξ = t − >0, the electric field is fully on. The overlap is a non-monotonic function of t n = nT . (Inset) The overlap at the end of the dynamical ramp tends to increase with increasing . Full size image Interestingly, for the parameters chosen, at t ≈ −11 T (that is, slightly before the electric field is fully on) the Bott index jumps from zero and becomes one, indicating the wavefunction has acquired a topological character. We also note that the overlap with the Floquet ground state increases non-monotonically with time. This suggests that the final overlap can be increased by using more sophisticated ramping protocols. For example, by instantaneously quenching the amplitude of the electric field from its value when the overlap has a local maximum to its final value. In the inset in Fig. 3 , we plot the value of the overlap with the Floquet ground state at the end of the ramp, that is, , for different ramping times and observe that, as expected, it generally increases with increasing . We note that the system can become topological even if the ramp is not adiabatic and the overlap between and is small. To relate the dynamical behaviour of the non-equilibrium Bott index to the properties of H F , we first study the critical field E c ( N sites ) at which the Floquet Hamiltonian becomes topological. For each system size, we compute the exact Floquet Hamiltonian for many different values of the electric field and repeat the analysis in Fig. 2c . For weak electric fields, Bott( ɛ ) is identically zero, while for E > E c the Bott index is unity for some energies. This allows us to extract E c for different system sizes, which is reported in Fig. 4a . A fit to those results shows that E c approaches the infinite system size result exponentially in the linear dimension of the system . The infinite size result is, in turn, compatible with the value =3.485 at which the translationally invariant system becomes topological, as shown by the Chern number of the lowest Floquet band in Fig. 4b . Next, we study the value of the electric field at the time at which the non-equilibrium Bott index jumps, that is, . One could advance that, when the driving is turned on very slowly (that is, adiabatically) is identical to E c ( N sites ) for any given system size. This is indeed what we find. In Fig. 4c , we show the critical field at which becomes topological, for a system with 928 sites, as a function of the ramping time. A fit to the results shows that approaches the adiabatic limit (infinite time ramp) result exponentially in the ramp time. Our extrapolated result for the adiabatic limit is compatible with E c ( N sites =928)≈5.0 for which H F becomes topological (see point signalled by an arrow in Fig. 4a ). We have also studied what happens if one fixes the ramp time and increases the system size, see Fig. 4d . In this case, the critical field approaches the thermodynamic limit result also exponentially with the linear dimension of the system. To make closer contact with experiments (such as ref. 17 ), we investigate the current that flows through the sample under driving ( Supplementary Fig. 2 and Supplementary Note 3 ). This is, in principle, a measurable quantity [24] . We stress that the physical current is different from the current one obtains using the Floquet Hamiltonian [18] , [25] (see Methods). The former connects only nearest-neighbour sites, while the latter can flow between far away lattice sites if there are longer-range hopping terms in H F . We compute the physical current by solving the time-dependent Schrödinger equation. Contrary to the overlap, the average current over a period continues to evolve for t > (that is, when the electric field amplitude has already reached its final value). Therefore, after the end of the ramp, we evolve the system for a large number of periods (10 3 ) so that the averaged current (over a period) becomes stationary. (We note that the instantaneous current still changes within a period.) Results for the average current are shown in Fig. 5 . Remarkably, we find that the chirality of the non-equilibrium current depends on the filling fraction (recall that the initial state is the ground state of H S ), see Supplementary Figs 3–7 and Supplementary Note 4 . To identify what changes when the Bott index jumps in systems at half filling, we have compared the currents for four different ramps ( Supplementary Figs 8 and 9 , Supplementary Table 1 and Supplementary Note 5 ). The first three ramps (last ramp) are (is) such that the final value of the electric field is smaller (larger) than the critical value required for the Bott index to jump. For the last ramp, after the Bott index jumps to one, the currents are much larger than for the first three ramps and are localized along the edges of the system. 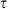Figure 5: Time-averaged physical current after a dynamical ramp with=80. We show results for systems with filling factors:ν=0.46, 0.5 and 0.54. The red colour indicates a current flowing from sublatticetoalong the nearest-neighbour vectorsδi:,δ3=a(−1, 0). The blue colour indicates the opposite direction. The black arrows indicate the direction of the edge current and are a guide to the eye. (a) For an initial fillingν=0.46, the non-equilibrium current is concentrated along the edges and moves anticlockwise. (c) For an initial fillingν=0.54, the non-equilibrium current is concentrated along the edges and moves clockwise. (b) At half filling, both chiralities are presents. On the top and left edge the current moves clockwise, while on the bottom and right edge it moves anticlockwise. These edge currents are balanced by a current diffusing through the bulk. The non-equilibrium wavefunctions corresponding toaandcare topologically trivial (Bott index is zero) while the one corresponding tobis topological non-trivial (Bott index is one). Figure 5: Time-averaged physical current after a dynamical ramp with =80. We show results for systems with filling factors: ν =0.46, 0.5 and 0.54. The red colour indicates a current flowing from sublattice to along the nearest-neighbour vectors δ i : , δ 3 = a (−1, 0). The blue colour indicates the opposite direction. The black arrows indicate the direction of the edge current and are a guide to the eye. ( a ) For an initial filling ν =0.46, the non-equilibrium current is concentrated along the edges and moves anticlockwise. ( c ) For an initial filling ν =0.54, the non-equilibrium current is concentrated along the edges and moves clockwise. ( b ) At half filling, both chiralities are presents. On the top and left edge the current moves clockwise, while on the bottom and right edge it moves anticlockwise. These edge currents are balanced by a current diffusing through the bulk. The non-equilibrium wavefunctions corresponding to a and c are topologically trivial (Bott index is zero) while the one corresponding to b is topological non-trivial (Bott index is one). Full size image The two topological invariants studied here during the switching on of a periodic perturbation, the Chern number in translationally invariant (thermodynamically large) systems and the Bott index in systems with boundaries, exhibit qualitatively different behaviour. The Chern number is conserved while the Bott index can change under unitary evolution. The conservation of the Chern number might appear surprising since, during any non-equilibrium process, some excitations are generated and the final state, which corresponds to a partially filled valence and conductance band, need not have a quantized Chern number. However, this argument does not take into account that under unitary evolution each quasi-momentum k is in a coherent superposition of the valence and conduction band. It is precisely this coherence that prevents the Chern number from changing. Our results for the Bott index show that, when one turns on a drive slowly starting from a topologically trivial state in finite systems with open boundary conditions, there is a critical field (which depends on the ramp time ) at which the Bott index jumps from zero to one. This indicates that the system becomes topologically non-trivial, even if the turn on is not adiabatic. If the drive is turned on adiabatically, approaches (with increasing system size) =3.485 at which the Chern number indicates that the Floquet Hamiltonian of the system with periodic boundary conditions becomes topological in the thermodynamic limit. This agrees with the intuition that an adiabatic turn on of the drive should allow one to generate a topologically non-trivial state, but is in stark contrast with the fact that the Chern number is a conserved quantity. Two possible explanations to these fundamental differences in thermodynamically large systems are: either dynamical topological transitions only occur in systems with boundaries or those transitions can happen in systems with and without boundaries, despite the fact that the Chern number does not change in the latter. Unfortunately, we have not been able to use the Bott index to discriminate between those possibilities. We note that the Bott index is not a smooth function of the energy in clean system with periodic boundary conditions ( Supplementary Fig. 10 and Supplementary Note 6 ). Closer to experiments, our results for the chiralities of the edge currents, namely, that they depend on the filling fraction, might also appear intriguing. They contrast with the fact, which we have checked, that the edge modes of a topological Floquet Hamiltonian support a single-particle current whose chirality is determined by the polarization of the electric field. Our results are a consequence of the fact that the current in many-particle non-equilibrium states has contributions from Floquet eigenstates with many different quasi-energies. While it is well known that a topological Floquet Hamiltonian supports chiral edge modes in the bulk gap, we have verified that other Floquet eigenstates can support currents with both the chiralities ( Supplementary Figs 3–7 and Supplementary Note 4 ). By changing the filling fraction one can change the contributions of different Floquet eigenstates and control the chirality of the resulting current. This means that any potentially sharp signature of the topological transition (identified by the jump in the Bott index) in the many-particle current is smeared out by the contributions of Floquet eigenstates that are away from the bulk gap. The dependence of the chirality on the filling fraction is a strong prediction of this work that can be tested in current experimental setups. Our results open many interesting questions: what is the nature of the topological transition in systems with boundaries? What is the dynamics of the edge states [26] across those transitions? What happens in the presence of interactions [27] , [28] and/or a coupling to a bath? Which loading protocols maximize the occupation of the Floquet ground state? What are the distinctive signatures of non-topological wavefunctions evolving according to topological Hamiltonian (and vice versa)? Is the presence of deep lying current carrying Floquet eigenstates connected to the existence of new topological invariants unique to Floquet systems? Which physical observables capture best the time change of the Bott index? Is there a dynamical topological transition in clean systems with periodic boundary conditions? If so, which topological indicator captures it? We hope our work will motivate further studies to address these and other related questions and to establish, in full mathematical rigor, the properties of the non-equilibrium Bott index introduced here. Chern number conservation under unitary evolution By going to momentum space, the system is parametrized as in equation (6), where S k and B k are three-dimensional time-dependent vector fields. The Chern number of the occupied state is simply the number of wrapping of the pseudo-spin configuration around the Bloch sphere (equation (7)). The exact equation of motion is equation (8) (we have set =1). Putting together equations (6) and (8), we can perform the calculation using standard manipulations of classical vector fields. Our results are, however, fully quantum. We now compute t Ch: where we have introduced the short-hand notation kx S = x S = S x , ky S = y S = S y , and we have suppressed the suffix k in S k . We consider the three terms separately: where we have used the evolution equation t S = S × B and the Binet–Cauchy identity: The second and third terms are more involved. For example: where we have used the distribution property of the cross product x ( S × B )= S x × B + S × B x . One can apply the Binet–Cauchy identity to obtain: In a similar way, we get: Putting all together, and carrying out the cancellations, we get: So far this expression is completely general. Now we use that the initial state is a pure state: from which it follows that S ˙ S =1, that is, S is a unit vector for any point in the Brillouin zone. We then observe that: Therefore, we arrive at equation (10) in the main text. We observe that: If the vector field B is smooth the mixed derivative commute, that is, B x , y = B y , x , and we arrive at: If x ( B y ˙ S ) and y ( B x ˙ S ) are continuous, we can use the periodicity of B and S in the Brillouin zone to obtain: We note that, up to this point, we have simply shown that ( t )=0 if S ( t ) and B ( t ) are sufficiently smooth and S ( t ) represents a pure state, that is, S ˙ S =1. However, to prove that the Chern number is conserved at all times, we still need to prove that, under time evolution (i) a pure state remains pure and (ii) a smooth pseudo-spin configuration remains smooth. To verify that this is indeed the case, we look into the equation of motion (8). We note that, under this equation, the length of the vector S is conserved, that is, t ( S ˙ S )=0, and therefore the condition (i) is verified. We also note that the equation of motion is a linear differential equation. If S ( t =0) is smooth in k x , k y and B ( t ) is smooth in k x , k y then S ( t ) remains smooth at all times. Therefore, the condition (ii) is verified. This concludes the proof of the theorem. The statement that the Chern number cannot change independently of the time evolution considered is similar to the result that, under unitary evolution, the von Neumann entropy is conserved. Both results do not predict the exact wavefunction at the end of a dynamical process but constrain the possible outcomes. Bott index for out-of-equilibrium systems Consider a single-particle Hamiltonian (defined by a matrix H ) on a lattice. Given the two diagonal matrices X i , j = x i δ i , j and Y i , j = y i δ i , j , where x i and y i are the coordinates of the i th lattice site, we defined two unitary matrices: where L x , y are the linear dimensions of the system. Let R be the projector onto the eigenstates with up to energy ɛ , that is, . In equilibrium, the Bott index at energy ɛ is defined as [15] : where and are the matrices U x and U y projected onto the states up to energy ɛ . In ref. 15 , the Bott index was defined on a torus geometry (that is, for H with periodic boundary conditions). We generalize the Bott index to other geometries and non-equilibrium situations by properly modifying the projector R . For example, one can change the boundary conditions in H from periodic to open by switching off some hopping elements. Using the projector constructed with the eigenstates of H with open boundary conditions in equation (27), one can compute the Bott index in a patch geometry. We further generalize the Bott index to non-equilibrium situations by taking into account the occupation of the states during the dynamics. The Bott index of the occupied states is obtained by replacing the matrices and with the matrices U x ( t ) and U y ( t ): where R ( t ) is the projector onto states occupied at time t . For example, if one has at t =0, at time t the projector becomes , where and are the time-evolved states. One expects the generalized Bott index to be quantized if R is a sufficiently local projector [15] , that is, R i , j is small if sites i and j are far from each other. Strong numerical evidence supporting the expectation that the non-equilibrium Bott index defined on the patch geometry is quantized is provided in the main text. However, we stress that a mathematically rigorous proof is lacking at the moment. On the other hand, the Bott index in clean systems (the systems in ref. 15 had disorder) on a torus is neither quantized nor a smooth function of the energy ( Supplementary Note 6 ). We expect this to be because the eigenstates of H for this problem are plane waves, which are non-local in real space. Currents To identify the current operator, we look into the time derivative of the site occupations: The equation of motion of c l is , where we have used the fact that any non-interacting fermionic Hamiltonian can be written as: . Similarly, we compute . Substituting these expressions in equation (29), and computing the expectation value, one obtains: where indicates the imaginary part, and we have used that and and the overline indicates complex conjugation. The continuity equation relates the time derivative of the local density to the net current: . This allows us to identify the current flowing from site m to site l as: It is crucial that the Hamiltonian that appears in the equation of motion and in the definition of the current is the time-dependent Hamiltonian H ( t ) and not the Floquet Hamiltonian H F . In general, the matrix elements of H ( t ) and H F are different. Hence, the current computed using the Floquet Hamiltonian is, in general, not equal to the current that will be measured in experiments [18] , [25] . For graphene subjected to circularly polarized electric field, H ( t ) contains only nearest-neighbour terms. This leads to a current flowing only between nearest-neighbour lattice sites, while H F contains longer range hopping, which lead to a current flowing between distant sites. In general, the exact current J m → l is time dependent because both the matrix element H l , m and the expectation value are time dependent. Moreover, in non-equilibrium situations, the site occupancies are non-stationary . This implies that the instantaneous current is not locally conserved, that is, . We have averaged the instantaneous current over a full driving period to obtain , which is approximately conserved, that is, . Numerical simulations for system with boundaries The time-dependent Hamiltonian is given by equation (2). Because of its non-interacting character, this problem can be efficiently solved in the single-particle basis [22] , [23] . We denote as H S and H 1 ( t ) the N sites × N sites matrices ( N sites being the number of lattice sites) that represent the static and time-dependent parts of the Hamiltonian in real space. The evolution operator over a cycle is given by: where and U ( t j +1 , t j ) is computed using a second-order Trotter–Suzuki decomposition [29] , [30] , [31] : Since H S is time independent, needs to be computed only once (this is done by diagonalizing H S ). This leaves the computation of , from the already diagonal H 1 ( t ), to be computed at each time step. By exact diagonalization of U ( T , 0), we obtain the Floquet eigenstates and eigenvalues: from which the single-particle Floquet Hamiltonian can be explicitly built as where We note that this procedure is not limited to high-frequency driving and gives the numerically exact Floquet Hamiltonian H F . The time discretization δt is chosen small enough to ensure that it does not affect the results. The lowest-energy single-particle eigenstates of H F ( H S ) are then collected into a rectangular matrix W F ( W S ) of size N sites × N p , where N p is the number of particles in the ground state (at half filling N p = N sites /2). For the parameters chosen (equation (5)) the Floquet phases θ l do not span the entire range [− π , π ] and therefore an unambiguous separation of the states in the ‘Floquet valence band’ and ‘Floquet conduction band’ is possible. The time evolution of the many-particle system is obtained by multiplying the matrix W S from the left with the square matrix U ( T , 0) of size N sites × N sites . The overlaps between many-particle wavefunctions can also be easily computed as determinants of products of matrices such as W F and W S , and their adjoints [22] , [23] . Moreover, the elements of the equal-time single-particle density matrix are given by the i , j element of the square matrix of size N sites × N sites . Non-stroboscopic times We have also computed wavefunctions overlaps and the Bott index at non-stroboscopic times. The overlap between the time-evolving state and the Floquet Fermi sea does not change after the electric field is fully on, with the Floquet Hamiltonian computed from U ( t + T , t )=exp[− iH F [ t ] T ]. (Note that the Floquet Hamiltonian depends on the choice of the initial time of period. However Floquet Hamiltonians corresponding to different choices of the initial time are unitary equivalent to each other, see for example, ref. 18 .) We also find that for all the Bott index does not change with time, that is, . Here is the first stroboscopic times at which the Bott index becomes unity. However, we found that just before the transition, in our case for times , the Bott index at non-stroboscopic times can jump back and forth between zero and one. This is similar, and probably related, to the oscillations observed in the (equilibrium) Bott index as the Fermi energy enters in the bulk gap ( Fig. 2c ). How to cite this article: D’Alessio, L. & Rigol, M. Dynamical preparation of Floquet Chern insulators. Nat. Commun. 6:8336 doi: 10.1038/ncomms9336 (2015).